A role for Bicaudal-D2 in radial cerebellar granule cell migration Bicaudal-D (BICD) belongs to an evolutionary conserved family of dynein adaptor proteins. It was first described in Drosophila as an essential factor in fly oogenesis and embryogenesis. Missense mutations in a human BICD homologue, BICD2, have been linked to a dominant mild early onset form of spinal muscular atrophy. Here we further examine the in vivo function of BICD2 in Bicd2 knockout mice. BICD2-deficient mice develop disrupted laminar organization of cerebral cortex and the cerebellum, pointing to impaired radial neuronal migration. Using astrocyte and granule cell specific inactivation of BICD2, we show that the cerebellar migration defect is entirely dependent upon BICD2 expression in Bergmann glia cells. Proteomics analysis reveals that Bicd2 mutant mice have an altered composition of extracellular matrix proteins produced by glia cells. These findings demonstrate an essential non-cell-autonomous role of BICD2 in neuronal cell migration, which might be connected to cargo trafficking pathways in glia cells. The Bicaudal-D ( BicD ) gene was initially identified in Drosophila based on dominant mutations that induce mirror-image pattern duplications along the anteroposterior axis, thereby giving rise to bicaudal embryos [1] . It was later established that the BICD protein facilitates dynein-mediated transport and is involved in the proper localization of posterior mRNA in Drosophila embryos [2] , [3] . In mammals two homologues of Bicaudal-D are present, named BICD1 and BICD2, which associate with microtubule minus-end-directed motor dynein [4] , [5] and various cargos, such as the nuclear envelope [6] and Rab6 secretory vesicles [7] . One currently favoured hypothesis is that BICD family members are adaptor proteins involved in microtubule-based transport by docking the dynein motor proteins to appropriate cargos [8] , [9] , [10] . Recently, mutations in BICD2 have been linked to a spectrum of motor neuron disorders, in particular, a dominant mild early onset form of SMA [11] , [12] , [13] , suggesting that BICD2 plays an important role in the nervous system. To further examine the in vivo function of BICD2, we generated Bicd2 knockout (KO) mice. Here we report that these mice develop defects in laminar organization of the cerebral cortex, hippocampus and cerebellar cortex, indicative of radial neuronal migration defects. Cell-specific inactivation of BICD2 in astrocytes and neuronal precursors revealed that radial cerebellar granule cell migration is non-cell-autonomous and intrinsic to cerebellar Bergmann glia cells. Mass spectrometry analysis revealed that Bicd2 mutant mice have strongly reduced levels of the extracellular matrix protein Tenascin C. Our data demonstrate that Bergmann glia cells provide critical cues for granule neuron polarization and migration, and that BICD2 is a critical part of the Bergmann glia signalling mechanism responsible for granule cell migration. This study reveals an unexpected action of BICD2 in glia cell-guided granule cell migration that is of key importance for cerebellar development and function. BICD2 is required for cerebral cortex development To generate an inducible Bicd2 KO allele, we introduced two resistance markers by sequential rounds of homologous recombination. In the first round, a neomycin cassette surrounded by loxP sequences was inserted into intron 1. In the second round, a puromycin selection marker, surrounded by loxP sequences and followed by a β-galactosidase (lacZ) reporter gene fused to a nuclear localization signal, was inserted downstream of the mouse Bicd2 gene ( Supplementary Fig. 1 ). Embryonic stem (ES) cells with this floxed Bicd2 allele (termed Bicd2 f ), were transfected with a plasmid expressing Cre recombinase yielding a KO Bicd2 ( Bicd2 − ) allele, that generates a transcript consisting of exon 1 of Bicd2 and the lacZ reporter gene ( Supplementary Fig. 1 ). Bicd2 f ES cell clones were used to generate mice carrying the inducible and KO Bicd2 alleles ( Supplementary Fig. 1A ). Matings between heterozygous Bicd2 +/− mice yielded Bicd2 −/− mice at near-Mendelian frequencies, but Bicd2 −/− mice displayed increased mortality during early post-natal life resulting in a sub-Mendelian frequency of Bicd2 −/− mice (13% of 208 mice) at P10. Late embryonic and newborn Bicd2 −/− mice were indistinguishable in gross appearance and weight from heterozygous and wild-type littermates ( Fig. 1a ), but after birth the Bicd2 −/− mice developed an enlarged dome-shaped skull, indicative of hydrocephalus ( Fig. 1b ). By P14 Bicd2 −/− mice started to show reduced weight compared with their littermates ( Fig. 1c ), and by P30 all Bicd2 −/− mice died. Behaviourally, Bicd2 −/− mice at P20 displayed motor abnormalities: the mice walked with an abnormal wide-based gait of both fore- and hindpaws, and frequently made missteps when placed on a grid ( Supplementary Movie 1 ). Furthermore, at 3 weeks of age, the mice were unable to walk on a balance beam and showed clasping rather than extension of the hindlimbs when lifted by their tail. 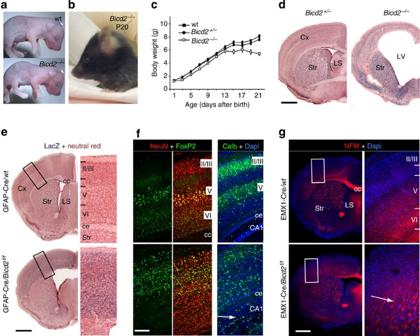Figure 1: Hydrocephalus and disrupted laminar organization of the cortex in BICD2-deficient mice. (a,b) Photographs of BICD2 KO (Bicd2−/−) mice showing a normal gross appearance at embryonic day 19 (a), and a dome-shaped head indicative of hydrocephalus at post-natal day 20 (b). (c) X–Y plot of body weight (mean±s.e.,n>4 per group) showing near-normal weight ofBicd2−/−mice up to post-natal day 13, and weight loss during subsequent days. (d) Coronal brain sections of P20 mice stained for LacZ and neutral red reveal enlarged lateral ventricles (LV), thinning of the cortex (Cx) and atrophy of several telencephalic areas including striatum (Str) and lateral septum (LS) in homozygoteBicd2−/−and no change in heterozygoteBicd2+/−mice. Note the moderate and high level of LacZ staining throughout the forebrain ofBicd2+/−andBicd2−/−mice, respectively, indicative of widespread BICD2 expression. (e) Coronal LacZ/neutral red-stained sections of the cortex of floxedBicd2f/fcrossed with aGFAP-Creline; the high magnification of the primary somatosensory cortex illustrates disrupted cortical laminar organization. Also note the thin corpus callosum (cc) and capsula externa (ce) inGFAP-Cre/Bicd2f/fmice. (f) Immunofluorescence of NeuN and FoxP2 or Calbindin showing altered laminar distribution of FoxP2 and calbindin inGFAP-Cre/Bicd2f/fcortex. FoxP2 that in control mice is present in lamina V and VI pyramidal neurons, inGFAP-Cre/Bicd2f/fcortex is distributed in superficial lamina. Note the absence of a laminar organization of NeuN+ cellsGFAP-Cre/Bicd2f/fcortex. Also note disorganized pyramidal cell layer in the CA1 ofGFAP-Cre/Bicd2f/fhippocampus (arrow). (g) Immunofluorescence of neurofilament-M (NFM) showing abnormally oriented axonal bundles coursing from the superficial lamina towards the capsula interna in neocortex ofEMX1-Cre/Bicd2f/fmice (arrow). Scale bars: 5 mm (a,b), 1 mm (d,e,g), 200 μm (e,f,g). Figure 1: Hydrocephalus and disrupted laminar organization of the cortex in BICD2-deficient mice. ( a , b ) Photographs of BICD2 KO ( Bicd2 −/− ) mice showing a normal gross appearance at embryonic day 19 ( a ), and a dome-shaped head indicative of hydrocephalus at post-natal day 20 ( b ). ( c ) X–Y plot of body weight (mean±s.e., n >4 per group) showing near-normal weight of Bicd2 −/− mice up to post-natal day 13, and weight loss during subsequent days. ( d ) Coronal brain sections of P20 mice stained for LacZ and neutral red reveal enlarged lateral ventricles (LV), thinning of the cortex (Cx) and atrophy of several telencephalic areas including striatum (Str) and lateral septum (LS) in homozygote Bicd2 −/− and no change in heterozygote Bicd2 +/− mice. Note the moderate and high level of LacZ staining throughout the forebrain of Bicd2 +/− and Bicd2 −/− mice, respectively, indicative of widespread BICD2 expression. ( e ) Coronal LacZ/neutral red-stained sections of the cortex of floxed Bicd2 f/f crossed with a GFAP-Cre line; the high magnification of the primary somatosensory cortex illustrates disrupted cortical laminar organization. Also note the thin corpus callosum (cc) and capsula externa (ce) in GFAP-Cre / Bicd2 f/f mice. ( f ) Immunofluorescence of NeuN and FoxP2 or Calbindin showing altered laminar distribution of FoxP2 and calbindin in GFAP-Cre/Bicd2 f/f cortex. FoxP2 that in control mice is present in lamina V and VI pyramidal neurons, in GFAP-Cre / Bicd2 f/f cortex is distributed in superficial lamina. Note the absence of a laminar organization of NeuN+ cells GFAP-Cre / Bicd2 f/f cortex. Also note disorganized pyramidal cell layer in the CA1 of GFAP-Cre / Bicd2 f/f hippocampus (arrow). ( g ) Immunofluorescence of neurofilament-M (NFM) showing abnormally oriented axonal bundles coursing from the superficial lamina towards the capsula interna in neocortex of EMX1-Cre/Bicd2 f/f mice (arrow). Scale bars: 5 mm ( a , b ), 1 mm ( d , e , g ), 200 μm ( e , f , g ). Full size image Examination of Bicd2 −/− mice at P15–P25 revealed no gross alterations in internal organs, except for a smaller size, and confirmed that Bicd2 −/− mice developed severe hydrocephalus, which was characterized by progressive expansion of lateral ventricles (ventriculomegaly), loss of white matter and ependymal cells surrounding the ventricles, severe thinning of the cortex and atrophy of other telencephalic areas, including striatum, hippocampus and septum ( Fig. 1d ; Supplementary Fig. 2A–D ). Apart from cerebellar cortex (see below), other brain regions and spinal cord appeared normal ( Supplementary Fig. 2F ). Analysis of the aqueduct at P5 suggested a smaller diameter indicative of aqueductal stenosis ( Supplementary Fig. 2E ). In addition to the Bicd2 −/− mice which completely lack the gene in all tissues, we generated mice that were deficient in BICD2 in the entire nervous system but showed normal BICD2 expression in most internal organs by crossing floxed Bicd2 f/f mice with Nestin-Cre mice [14] . Nestin-Cre Bicd2 f/f mice reproduced the severe progressive hydrocephalus, neurological features and short lifespan of Bicd2 −/− mice ( Table 1 ). Crossing of Bicd2 f/f mice with GFAP-Cre mice, which exhibit sustained Cre-recombinase expression in astrocytes and transient Cre activity in some neuronal precursor cells [15] , resulted in less severe or no hydrocephalus ( Table 1 ). GFAP-Cre Bicd2 f/f mice without hydrocephalus revealed a second major nervous system abnormality of BICD2-deficient mice, that is, a disordered laminar organization of the cerebral cortex ( Fig. 1e ) and hippocampus ( Supplementary Fig. 3 ). Consistent with impaired radial migration, Foxp2, a marker predominantly found in deep corticofugal layer V and VI neurons, was present in superficial layers in GFAP-Cre Bicd2 f/f mice ( Fig. 1f ). Corticofugal axonal trajectories (labelled with anti-neurofilament M antibody) arose in superficial instead of deep cortical layers. Importantly the same cortical and hippocampal phenotype was also observed in EMX1-Cre Bicd2 f/f mice that are selectively deficient for BICD2 in radial glia, glutamatergic neurons and astrocytes in the cortex and hippocampus [16] ( Table 1 ; Fig. 1g ). Together, the data from GFAP-Cre and EMX1-Cre Bicd2 f/f mice indicate that BICD2 is essential for the proper development of the cerebral cortex, and suggest that BICD2 plays a role in radial migration of excitatory neurons. These data are consistent with the neurogenesis and early neuronal migration defects observed after BICD2 knockdown in cortical brain slices by in utero electroporation [17] . Table 1 Principal features of ubiquitous and region-specific BICD2-deficient mice used in this study. Full size table BICD2 is required for cerebellar granule cell migration In the cerebral cortex, radial glia progenitor cells give rise to neurons and glia cells and act as a scaffold for radial migration, making it difficult to differentiate between potential glia- and neuron-specific defects and to decipher to which extent disorganized laminar organization follows from neurogenesis abnormalities or impaired migration [18] . In the cerebellar cortex, however, granule cells originate in the external granule cell layer (EGL) and migrate inward to the internal granule cell layer (IGL) along radial processes of Bergmann glia. Granule and glial cells originate from different precursors [19] , [20] , which makes it easier to establish the origin of migration deficits. Bicd2 −/− mice showed a disproportionally small cerebellum with grossly intact subdivision in vermis and hemispheres and foliation ( Fig. 2a ; Supplementary Fig. 2 ), but an altered laminar organization, indicative of the absence of radial granule cell migration. Instead of laminar subdivision into molecular, Purkinje cell and granular layer, in Bicd2 −/− cerebellar cortex the cell bodies of Purkinje cells (Calbindin+, NeuN−) were positioned near the white matter, while other neurons (NeuN+) were spread over a single superficial layer ( Fig. 2b,c ). This layer contained both molecular layer interneurons (NeuN+, Parvalbumin+, Calbindin−), as well as a high density of granule cells, identified by immunostaining for the α6 GABA A receptor subunit that is only expressed by adult, post-migratory granule cells ( Fig. 2d–g ). Cerebellar Golgi cells (mGluR2+), which are localized in the granule cell layer of wild-type mouse cerebellar cortex, were concentrated between the white matter and the Purkinje cell layer, and did not occur in Bicd2 −/− molecular/granule cell layer ( Supplementary Fig. 4 ). Staining for the glutamate synaptic vesicle transporter VGluT1, which is present in parallel fibre and mossy fibre endings in the cerebellar molecular and granular layers, respectively, revealed prominent punctate staining in the Bicd2 −/− molecular/granular layer, indicative of the presence of parallel fibre endings ( Fig. 2f,g ). VGluT1-immunostaining near the Purkinje cell layer also revealed sporadic larger irregular structures resembling mossy fibre endings, which accordingly co-distributed with α6 GABA A receptor immunoreactivity, indicative of granule cell dendritic processes in the glomeruli ( Fig. 2g ). Immunostaining for VGluT2, which is present in an additional and partially overlapping population of mossy fibre endings as well as in climbing fibre endings, confirmed the presence of a low number of mossy fibre endings and indicated impaired climbing fibre innervation of Purkinje cells in Bicd2 −/− cerebellar cortex ( Supplementary Fig. 4C,D ). Immunostaining for zebrin II suggests preserved parasagittal compartmentalization of Purkinje cells ( Supplementary Fig. 4E,F ). 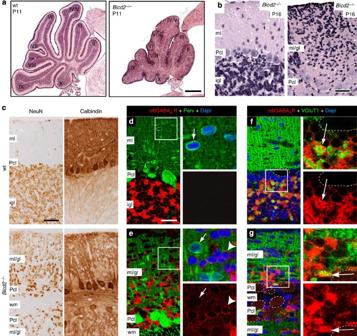Figure 2: Granule cells populate the molecular layer inBicd2−/−cerebellar cortex. (a,b) Sagittal sections of P11 and P16 cerebellum stained with H&E. The low magnification inaillustrates the intact folial organization of the vermis ofBicd2−/−cerebellar cortex. The high magnification inbshows the absence of the internal granule cell layer (igl) and a high density of cells in the molecular layer (ml) inBicd2−/−cerebellum. (c) Sagittal sections of P16 cerebellum immunostained with anti-NeuN and anti-calbindin. Note that inBicd2−/−cerebellar cortex the Purkinje cell layer (Pcl, calbindin+ cells) is localized adjacent to the white matter (wm), and that Purkinje cell dendritic arbors extend up to the pial surface. (d–g) Double-labelling confocal immunofluorescence of α6 GABAAreceptor subunit (α6GABAAR) with parvalbumine (Parv) and VGluT1, respectively, in transverse sections of P20 cerebellum. Note the presence of many α6GABAAR+ cells (arrow head ine), a moderate amount of Parv+ cells (arrow ine), and abundant VGluT1 labelling (g) in the ml/gl layer ofBicd2−/−cerebellar cortex. The arrow infpoints to a glomerulus containing both α6GABAAR+ granule cell dendritic processes and a VGluT1+ mossy fibre ending. Occasionally, double-labelled glomeruli-like structures occur near the Pcl ofBicd2−/−cerebellar cortex (arrow ing). Optical sections ind–g, 1 μm. Scale bars: 200 μm (a), 25 μm (b,d), 50 μm (c). Figure 2: Granule cells populate the molecular layer in Bicd2 −/− cerebellar cortex. ( a , b ) Sagittal sections of P11 and P16 cerebellum stained with H&E. The low magnification in a illustrates the intact folial organization of the vermis of Bicd2 −/− cerebellar cortex. The high magnification in b shows the absence of the internal granule cell layer (igl) and a high density of cells in the molecular layer (ml) in Bicd2 −/− cerebellum. ( c ) Sagittal sections of P16 cerebellum immunostained with anti-NeuN and anti-calbindin. Note that in Bicd2 −/− cerebellar cortex the Purkinje cell layer (Pcl, calbindin+ cells) is localized adjacent to the white matter (wm), and that Purkinje cell dendritic arbors extend up to the pial surface. ( d – g ) Double-labelling confocal immunofluorescence of α6 GABA A receptor subunit (α6GABA A R) with parvalbumine (Parv) and VGluT1, respectively, in transverse sections of P20 cerebellum. Note the presence of many α6GABA A R+ cells (arrow head in e ), a moderate amount of Parv+ cells (arrow in e ), and abundant VGluT1 labelling ( g ) in the ml/gl layer of Bicd2 −/− cerebellar cortex. The arrow in f points to a glomerulus containing both α6GABA A R+ granule cell dendritic processes and a VGluT1+ mossy fibre ending. Occasionally, double-labelled glomeruli-like structures occur near the Pcl of Bicd2 −/− cerebellar cortex (arrow in g ). Optical sections in d – g , 1 μm. Scale bars: 200 μm ( a ), 25 μm ( b , d ), 50 μm ( c ). Full size image Analysis of early post-natal brain indicated that Bicd2 −/− cerebellar cortex appeared normal at post-natal day 2, before the onset of radial migration. As in control, the subsequent days was characterized by proliferation of granule cells and the gradual expansion of the area between the Purkinje cell layer and the pial surface. However, instead of migrating and forming the interior granule cell layer, granule cells accumulated throughout the molecular layer ( Fig. 3a,b ). Consistent with impaired inward radial migration, no granule cells with a polarized radially oriented elongated shape characteristic for migration [21] were present in the molecular layer of Bicd2 −/− P5–P15 cerebellar cortex ( Fig. 3c,d ). Thus, the absence of profiles of radially migrating cells, the accumulation of granule cells in the molecular layer and the absence of an IGL show that inward radial granule cell migration is severely disrupted in Bicd2 −/− mice ( Supplementary Movie 2 ). 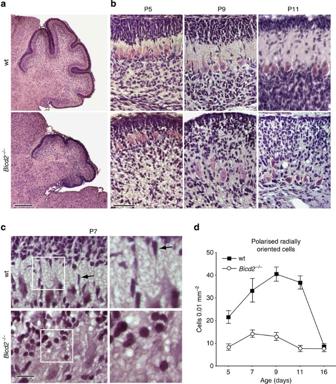Figure 3: No radial granule cell migration inBicd2−/−cerebellar cortex. (a–c) Sagittal paraffin sections of P5 (a,b), P7 (c), P9 and P11 section stained with H&E showing development ofBicd2−/−cerebellar cortex during the period of radial granule cell migration. Note the multiple flattened radially oriented cells in the nascent molecular layer of wild-type (arrows inbandc) but not inBicd2−/−cerebellar cortex. (d) Plot of density of flattened radially oriented cells (mean±s.e.,N=10) in the molecular layer (wt mice) or the mixed molecular/granular layer (Bicd2−/−) extending from the Purkinje cell layer up to 20 μm below the pial surface. Scale Bars: 200 μm (a), 50 μm (b), 20 μm (c). Figure 3: No radial granule cell migration in Bicd2 −/− cerebellar cortex. ( a – c ) Sagittal paraffin sections of P5 ( a , b ), P7 ( c ), P9 and P11 section stained with H&E showing development of Bicd2 −/− cerebellar cortex during the period of radial granule cell migration. Note the multiple flattened radially oriented cells in the nascent molecular layer of wild-type (arrows in b and c ) but not in Bicd2 −/− cerebellar cortex. ( d ) Plot of density of flattened radially oriented cells (mean±s.e., N =10) in the molecular layer (wt mice) or the mixed molecular/granular layer ( Bicd2 −/− ) extending from the Purkinje cell layer up to 20 μm below the pial surface. Scale Bars: 200 μm ( a ), 50 μm ( b ), 20 μm ( c ). Full size image BICD2 is expressed in Bergman glia but not in granule cells Analysis of BICD2 expression by western blotting showed the presence of BICD2 protein in multiple tissues including the brain. It also confirmed the absence of BICD2 in tissue homogenates from Bicd2 −/− mice and reduced expression in heterozygous Bicd2 +/− mice ( Fig. 4a , Supplementary Fig. 5 ). BICD2 is expressed at relatively high levels in embryonic and early post-natal brain, while its expression decreases after P10, resulting in relatively low levels in adulthood ( Fig. 4b , Supplementary Fig. 5 ). The absence of BICD2 in the KO mice did not lead to a significant change in the expression level of its close homologue BICD1 ( Fig. 4c ), indicating that there is no up- or downregulation of BICD1 in the absence of BICD2. Moreover, absence of BICD2 in the cerebellum and cortex did not change the expression levels of BICD2 binding partners, such as Rab6 and cytoplasmic dynein (DIC74) and its regulatory proteins dynactin (p150Glued) and Lis1 ( Fig. 4c , Supplementary Fig. 5 ). 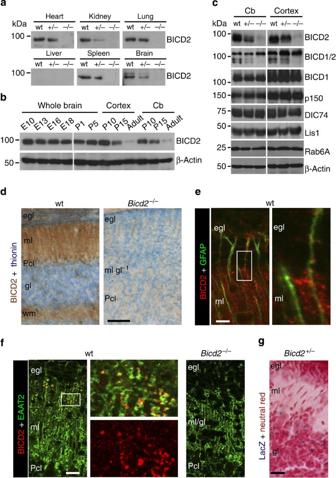Figure 4: Preferential BICD2 expression in Bergman glia in cerebellar cortex. (a) Western blot with BICD2 antibody (#2294) showing reduced and no expression of BICD2 in tissue homogenates of P20 heterozygoteBicd2+/−(+/−) and homozygoteBicd2−/−(−/−) mice, respectively. (b) Western blot showing relatively high BICD2 expression in developing nervous system. (c) Comparative western blot analysis showing unaltered BICD1 (antibody #2295 for BICD1, and upper band in strip stained with antibody #2293 for BICD1/2), dynein components and interacting proteins (dynactin p150, dynein intermediate chain 74, Lis1) and Rab6 expression inBicd2−/−cortex and cerebellum. Full-size western blots can be found inSupplementary Fig. 5. (d) Immunohistochemistry with anti-BICD2 antibody showing the absence of staining in P10Bicd2−/−cerebellar cortex and prominent staining in the molecular layer (ml) and the white matter (wm) of wild-type cerebellar cortex. (e,f) Double-labelling confocal immunofluorescence (optical sections 1 μm) showing co-distribution of BICD2 with GFAP and the excitatory amino-acid transporter EAAT2 in the ml and the egl. Note in right panel in (f) that EAAT2 labelling appears the same as in wild-type inBicd2−/−cerebellar cortex. (g) LacZ staining in sagittal cerebellar section of P10 heterozygoteBicd2+/−mice is predominantly present in the Purkinje cell layer. Scale Bars: 50 μm (d), 20 μm (f,g), 10 μm (e). Figure 4: Preferential BICD2 expression in Bergman glia in cerebellar cortex. ( a ) Western blot with BICD2 antibody (#2294) showing reduced and no expression of BICD2 in tissue homogenates of P20 heterozygote Bicd2 +/− (+/−) and homozygote Bicd2 −/− (−/−) mice, respectively. ( b ) Western blot showing relatively high BICD2 expression in developing nervous system. ( c ) Comparative western blot analysis showing unaltered BICD1 (antibody #2295 for BICD1, and upper band in strip stained with antibody #2293 for BICD1/2), dynein components and interacting proteins (dynactin p150, dynein intermediate chain 74, Lis1) and Rab6 expression in Bicd2 −/− cortex and cerebellum. Full-size western blots can be found in Supplementary Fig. 5 . ( d ) Immunohistochemistry with anti-BICD2 antibody showing the absence of staining in P10 Bicd2 −/− cerebellar cortex and prominent staining in the molecular layer (ml) and the white matter (wm) of wild-type cerebellar cortex. ( e , f ) Double-labelling confocal immunofluorescence (optical sections 1 μm) showing co-distribution of BICD2 with GFAP and the excitatory amino-acid transporter EAAT2 in the ml and the egl. Note in right panel in ( f ) that EAAT2 labelling appears the same as in wild-type in Bicd2 −/− cerebellar cortex. ( g ) LacZ staining in sagittal cerebellar section of P10 heterozygote Bicd2 +/− mice is predominantly present in the Purkinje cell layer. Scale Bars: 50 μm ( d ), 20 μm ( f , g ), 10 μm ( e ). Full size image Immunohistology shows that BICD2 is diffusely distributed throughout the nervous system. Relatively high staining intensities occurred in non-neuronal cells (NeuN−) and some populations of neurons (NeuN+), including motor neurons in cranial nerve motor nuclei and large neurons throughout the reticular formation ( Supplementary Fig. 6A–E ). The specificity of the staining for BICD2 was confirmed by the absence of staining in sections from Bicd2 −/− mice. In post-natal and adult cerebellar cortex, BICD2 immunoreactivity occurred in all layers, with the highest staining intensity in the molecular layer and the white matter ( Fig. 4d ). In the molecular layer, BICD2 immunoreactivity co-localized with GFAP and the excitatory amino-acid transporter EAAT2 (GLT1, SLCIA2) indicating that it is associated with Bergmann glial cells ( Fig. 4e,f ). No staining above background was observed in Purkinje cells and pre- and post-migratory granule cells in the EGL and IGL, respectively. The preferential labelling of BICD2 in Bergmann glia is in agreement with in situ hybridization data from the Allen Mouse Brain Atlas [22] , and with the preferential distribution of LacZ staining in Bergmann glial cells in cerebellar cortex of heterozygous Bicd2 +/− mice ( Fig. 4g ). Furthermore, also in neuron-astrocyte cerebellar co-cultures BICD2 staining was present in GFAP-positive astroglial cells but not in MAP2-positive cells ( Supplementary Fig. 6F ). Taken together, our data indicate that BICD2 is not expressed in premigratory or migrating granule cells, but rather in Bergmann glial cells, which are essential for successful radial migration of granule neurons in the cerebellum. BICD2 has a non-cell-autonomous function in migration The predominant expression of BICD2 in Bergman glia cells raises the possibility that defects in radial granule cell migration in Bicd2 −/− mice result from the loss of BICD2 function in Bergmann glia. Accordingly, crossing of Bicd2 f/f mice with GFAP-Cre mice, which show sustained Cre-recombinase expression in astrocytes including Bergmann glia, results in the same granule cell migration defects that are observed in global Bicd2 −/− mice ( Fig. 5a ). However, in view of Cre activity in some neuronal precursor cells including cerebellar granule cells [15] , the data from GFAP-Cre/ Bicd2 f/f mice do not exclude a role of BICD2 in migrating granule cells. We therefore crossed Bicd2 f/f mice with Math1-CreERT2 mice, which express tamoxifen-inducible Cre-recombinase in granule precursor cells [23] , and injected pregnant mothers with tamoxifen. Math1-CreERT2 / Bicd2 f/f offspring showed a normal cerebellar cortex, and systematic analysis of sections stained for the post-migratory granule cell marker α6 GABA A receptor showed that all granule cells were in the IGL at P20 ( Fig. 5b ). This indicated that elimination of BICD2 in premigratory cells does not affect radial granule cell migration. To further exclude that BICD2 has a cell intrinsic role in migrating granule cells, we performed shRNA-mediated knockdown of BICD2 in premigratory granule cells using ex vivo electroporation of P10 rat cerebella. Consistent with the data from Math1-CreERT2 / Bicd2 f/f mice, radial granule cell migration was unaltered in BICD2 shRNA treated granule cells ( Fig. 5c ). These data indicate that cerebellar granule cell migration defects in Bicd2 −/− mice are non-cell-autonomous and intrinsic to astrocytes. 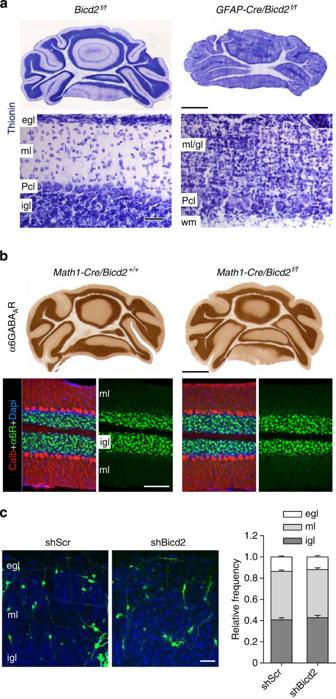Figure 5: BICD2 depletion in premigratory cerebellar granule cell does not influence radial migration. (a) Coronal thionin-stained sections showing that GFAP-Cre/Bicd2f/fdo not develop an IGL. (b) Unaltered distribution of α6GABAAR-labelled granule cells in P25Math1-CreERT2/Bicd2f/fcerebellar cortex. (c) P10 rat cerebella wereex vivoelectroporated withBicd2or scrambled control shRNAs and GFP expression vector. The fraction of GFP+ granule cells was quantified for each layer per picture (three separate experiments were performed, total number of pictures analysed for shScr=40, shBicd2=33). The average distribution of GFP+ granule cells is shown in the graph (error bars are s.e.m.,n=3). Scale bars: 1 mm (topa,b), 100 μm (b), 50 μm (a,c). Figure 5: BICD2 depletion in premigratory cerebellar granule cell does not influence radial migration. ( a ) Coronal thionin-stained sections showing that GFAP-Cre/ Bicd2 f/f do not develop an IGL. ( b ) Unaltered distribution of α6GABA A R-labelled granule cells in P25 Math1-CreERT2 / Bicd2 f/f cerebellar cortex. ( c ) P10 rat cerebella were ex vivo electroporated with Bicd2 or scrambled control shRNAs and GFP expression vector. The fraction of GFP+ granule cells was quantified for each layer per picture (three separate experiments were performed, total number of pictures analysed for shScr=40, shBicd2=33). The average distribution of GFP+ granule cells is shown in the graph (error bars are s.e.m., n =3). Scale bars: 1 mm (top a , b ), 100 μm ( b ), 50 μm ( a , c ). Full size image BICD2 does not influence Bergmann glial cell morphology All the results indicate that the radial granule cell migration deficit in Bicd2 −/− mice results from a loss of function of BICD2 in Bergmann glia, which has a scaffolding function in radial granule cell migration. It is thus conceivable that the disruption of Bergmann fibre scaffold causes the Bicd2 −/− cerebellar phenotype. GFAP immunohistochemistry showed that Bicd2 −/− mice show abundant radial glial fibre labelling ( Fig. 6a,b ). Bicd2 −/− radial glia showed an ordered radial organization of in the EGL with orthogonal orientation relative ( Fig. 6a–c ). In view of a small proportion of GFAP-positive fibres with abnormal non-radial orientation ( Fig. 6b ), we further analysed Bergmann glial cells in Bicd2 −/− mice crossed with GFAP–GFP transgenic mice that express GFP in a subset of Bergmann glial cells. Consistent with a grossly normal organization of Bergmann glia, the far majority of GFP-labelled Bergmann glia cells had the cell body near the Purkinje cells and radial processes extending up to the pial surface as in wild-type mice ( Fig. 6d–g ). These results indicate that morphology and structure of Bergmann glial cells are largely unaffected in Bicd2 −/− mice. 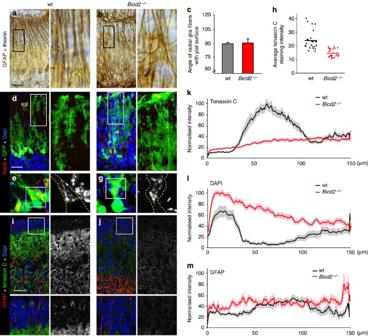Figure 6: Altered extracellular matrix composition in BICD2-deficient cerebellar cortex. (a,b) GFAP immunoperoxidase histochemistry in P10 coronal sections showing ordered radially oriented Bergmann glia processes in wild-type (wt) and more disorganized processesBicd2−/−cerebellum. (c) Quantification of the angle of the Bergmann glia cell radial processes with the pial surface (mean±s.e.,N=250) fromwtandBicd2−/−mice. (d–g) Maximal projection of confocal stack (11 sections, total thickness of optical section, 5 μm) of Rab6 immunofluorescence in coronal P20 cerebellar sections fromwtandBicd2−/−mice that also are transgenic for a GFAP-EGFP construct resulting in the expression of EGFP in subsets of astrocytes, including Bergmann glia cells. Note EGFP-positive Bergman glia cells that extend radial processes to the pial surface cerebellum in both wt (d) andBicd2−/−(f) cerebellum. Also note that Rab6 immunoreactivity which is mainly distributed in the trans-Golgi apparatus shows the same distribution inwtandBicd2−/−Bergman glia cell body (e,g). (h–j) Double-labelling confocal immunofluorescence (optical sections 1.5 μm) of tenascin and GFAP immunoreactivity showing reduced labelling inBicd2−/−cerebellum. (k–m) Fluorescent intensity of the indicated marker in the molecular layer (wt mice) or the mixed molecular/granular layer (Bicd2−/−mice) from the pial surface up to the Purkinje cell layer. Scale bars: 25 μm (a,d,i). Figure 6: Altered extracellular matrix composition in BICD2-deficient cerebellar cortex. ( a , b ) GFAP immunoperoxidase histochemistry in P10 coronal sections showing ordered radially oriented Bergmann glia processes in wild-type (wt) and more disorganized processes Bicd2 −/− cerebellum. ( c ) Quantification of the angle of the Bergmann glia cell radial processes with the pial surface (mean±s.e., N =250) from wt and Bicd2 −/− mice. ( d – g ) Maximal projection of confocal stack (11 sections, total thickness of optical section, 5 μm) of Rab6 immunofluorescence in coronal P20 cerebellar sections from wt and Bicd2 −/− mice that also are transgenic for a GFAP-EGFP construct resulting in the expression of EGFP in subsets of astrocytes, including Bergmann glia cells. Note EGFP-positive Bergman glia cells that extend radial processes to the pial surface cerebellum in both wt ( d ) and Bicd2 −/− ( f ) cerebellum. Also note that Rab6 immunoreactivity which is mainly distributed in the trans-Golgi apparatus shows the same distribution in wt and Bicd2 −/− Bergman glia cell body ( e , g ). ( h – j ) Double-labelling confocal immunofluorescence (optical sections 1.5 μm) of tenascin and GFAP immunoreactivity showing reduced labelling in Bicd2 −/− cerebellum. ( k – m ) Fluorescent intensity of the indicated marker in the molecular layer (wt mice) or the mixed molecular/granular layer ( Bicd2 −/− mice) from the pial surface up to the Purkinje cell layer. Scale bars: 25 μm ( a , d , i ). Full size image BICD2 −/− mice have altered extracellular matrix composition Having shown that migration defects in Bicd2 −/− mice are intrinsic to the Bergmann glial cells, we wanted to gain a better understanding of how BICD2 regulates cerebellar granule cell migration. We first focussed on the subcellular distribution of known BICD2 binding partners, such as Rab6, dynein/dynactin and RanBP2. Immunofluorescence with antibodies against these proteins revealed no major changes in Bicd2 −/− Bergmann glia ( Fig. 6e,g ). Moreover, no change in centrosome position or Golgi apparatus morphology was observed in these cells. Next, we searched for molecular changes in Bicd2 −/− mice using mass spectrometry. Proteomics analysis was performed with biological duplicates on cerebellar extracts from control and homozygote Bicd2 −/− mice at P15. Mass spectrometry analysis of whole lanes revealed several up- and downregulated proteins, and we decided to focus on the factors that were previously found to influence neuronal migration, including signalling factors, extracellular matrix and adhesion molecules [24] , [25] , [26] , [27] , [28] . Some of these proteins were only mildly affected in the Bicd2 −/− cerebellum, while others like N-cadherin and integrin β1 showed a strongly reduced expression ( Table 2 and Supplementary Data 1 ). Only two proteins were absent from the Bicd2 −/− cerebellum in two separate experiments, doublecortin (DCX) and Tenascin C. Since microtubule-associated protein DCX is restricted to migrating neurons and absent from Bergmann glia cells [29] , [30] , we further analysed the extracellular matrix protein Tenascin C. Tenascin C is produced by Bergmann glia cells [31] , has been implicated in neuron-glia cell recognition [32] , [33] and is known to be important for granule cell migration in the cerebellum [34] , [35] , [36] , [37] . We determined the Tenascin C distribution by immunofluorescence experiments using antibody staining and confirmed that the levels of Tenascin C in the Bicd2 −/− cerebellum were low ( Fig. 6h–j ). Thus while Tenascin C was abundantly present in the molecular layer of P7–P15 wild-type cerebellum, the levels of Tenascin C were low throughout the cerebellar cortex in Bicd2 −/− mice at this age ( Fig. 6i-m ). Together these data show that Bicd2 −/− mice have an altered extracellular matrix composition in the molecular layer, which could be responsible for the defects in granule cell migration. Table 2 Proteomics analysis from biological duplicates of cerebellar extracts from control and homozygote Bicd2 −/− mice at P15. Full size table In this study, we have shown that the conserved dynein adaptor protein BICD2 is essential for proper development of the brain, where it plays an important role in the establishment of the laminar organization of the cerebral and cerebellar cortices. In particular, by comparing different mouse lines missing BICD2 in specific cell populations, we demonstrated that BICD2 has a non-cell-autonomous function in driving inward radial migration of cerebellar granule cells. In addition, by using a proteomic approach we provide evidence that the extracellular matrix protein Tenascin C produced by the Bergmann glia cells may account for the non-cell-autonomous role of BICD2 in migration. Multiple factors have been identified that control granule cell migration in a cell-autonomous manner [24] , [25] , [26] , [27] , [28] , such as proteins that control centrosome positioning and nucleokinesis [38] , [39] , [40] , [41] and neuronal adhesion molecules that mediate granule cell-Bergmann glia interaction [42] , [43] , [44] . Moreover, several abnormalities in Bergmann glia cell structure and function have been shown to cause granule cell migration alterations [19] , [20] . For instance, mutant mice that disrupt the radial scaffold structure of Bergmann glia fibres develop migration deficits [45] , [46] , [47] . Also mutant mice with Bergmann glia fibres with abnormal end feet at the pial surface show impaired migration and develop clusters of ectopic granule cells [48] , [49] . An important feature of the Bicd2 −/− mice is the complete absence of an IGL, indicating a severe disruption of granule cell migration ( Supplementary Movie 2 ). This phenotype is more severe than the migration deficits found in any other granule cell migration deficient mouse model. In addition, the laminar distribution of other cerebellar cortical neurons including Purkinje cells and molecular layer interneurons appears intact, indicating that the migration deficit is specific for granule cells. Furthermore, only subtle abnormalities in the overall Bergmann glia cell organization are observed, suggesting that the granule cell migration deficit in Bicd2 −/− mice cannot be explained by structural changes in Bergmann glia morphology. Nevertheless, our data strongly indicate that the granule cell migration deficits result from a loss of function of BICD2 in Bergmann glia, as BICD2 is expressed in Bergmann glia cells, but not in premigratory or migrating granule cells. In addition, selective deletion of BICD2 in premigratory granule cells does not influence radial migration, while the depletion of BICD2 in astrocytes including Bergmann glia cells leads to the same granule cell migration defects as observed in global Bicd2 −/− mice. The data indicate that BICD2 has a non-cell-autonomous role in granule cell migration in the cerebellar cortex. How can BICD2 exert non-cell-autonomous effects? We envision two scenarios that are not mutually exclusive. First BICD2 could regulate dynein-mediated trafficking in Bergmann glia cells. BICD2 is a regulator of dynein function and plays a role in dynein-mediated cellular processes, such as microtubule minus-end-directed trafficking [3] . BICD2 binds to the dynein motor complex [4] , promotes a stable interaction between dynein and its assessory factor dynactin [50] and induces microtubule-dependent minus-end-directed transport [5] . Similar to the Drosophila BICD mutant embryos [2] , Bergmann glia cells lacking BICD2 could have defects in dynein-mediated transport pathways. However, we did not observe cellular phenotypes related to globally impaired dynein/dynactin function in Bergmann glia cells, such as Golgi fragmentation and other signs of impaired retrograde trafficking. Other dynein regulators, such as lissencephaly 1 (Lis-1) and nuclear distribution protein E (NDE1) have previously been found to control neuronal migration [38] , [41] . Second, it is possible that BICD2 is involved in a specific cargo trafficking pathway in Bergmann glia cells. For instance, BICD2 also interacts with the small GTPase Rab6, which controls the targeting and fusion of secretory vesicles to the plasma membrane [8] , [9] , [10] . However, very little is known about the trafficking and secretion mechanisms in Bergmann glia cells. On the basis of the involvement of BICD2 in secretory transport in other systems, we speculate that the trafficking or secretion of neuron–glial cell recognition factors might be altered in Bicd2 −/− mice. Indeed, the extracellular matrix protein Tenascin C produced by Bergmann glia cells is found at relative low levels in Bicd2 −/− mice. Tenascin C is known to mediate the attachment of neurons to astrocyte surfaces in in vitro cell binding assays and stimulates granule cell migration in the cerebellum [31] , [34] , [35] , [36] , [37] . It is interesting to note that the early neuronal migration and differentiation marker DCX is not detected in Bicd2 −/− cerebellum extracts, suggesting a potential link between extracellular matrix components and granule cell migration [51] . Our findings demonstrate an essential non-cell-autonomous role of BICD2 in neuronal cell migration, which might be connected to cargo trafficking pathways in Bergmann glia cells. BICD2-deficient mice also displayed a disordered laminar organization of the cerebral cortex and hippocampus, which is compatible with a deficit in radial outward migration of newly born neurons to the cortical plate. These data imply that BICD2 may also have a similar non-cell-autonomous function in cortical radial glia cells. However, in the cortex, radial glial cells also act as neuronal progenitor cells, making it difficult to differentiate between potential glia and neuron-specific defects. At least part of the laminar abnormalities can be explained by a recently identified role of BICD2 in cell-cycle-dependent nuclear oscillation in radial glial progenitors [17] . BICD2 recruits dynein to the nucleopore complex in G2 to mediate apical nuclear migration and BICD2 knockdown causes cell cycle arrest and neurogenesis deficits [6] , [17] . The extent to which different potential functions of BICD2 contribute to cortical and hippocampal migration deficits remains to be determined. Recently, mutations in BICD2 have been linked to a dominant mild early onset form of SMA [11] , [12] , [13] . The motor symptoms show congenital or early post-natal onset, are non-progressive and are associated with chronic muscle denervation and reinnervation, suggesting problems with maintaining the axon or the neuromuscular synapse. Spinal cord and motor neurons appeared normal in the Bicd2 −/− mice, and we did not observe any motor neuron abnormalities or signs of impaired retrograde transport defects. The differences in phenotypes between Bicd2 −/− mice and the SMA patients with mutations in BICD2 gene indicate that the motor neuron defects cannot be explained by the loss of BICD2 function. Indeed, a transgenic mouse expressing the N-terminal part of BICD2, which has a strong dynein-recruiting activity and chronically impaired dynein–dynactin function, develops several cellular phenotypes in motor neurons including Golgi fragmentation and neurofilament accumulation in the proximal axon [52] . These phenotypes are compatible with the pathology developed by patients. The missense BICD2 mutations found in SMA patients could thus exert a gain of function effect, consistent with the dominant character of the disease. Future studies are needed to further unravel the multiple essential roles of BICD2 in nervous system development. Animals All animal experiments were performed in compliance with the guidelines for the welfare of experimental animals issued by the Federal Government of The Netherlands. All animal experiments were approved by the Animal Ethical Review Committee (DEC) of the Erasmus Medical Center and Utrecht University. The BICD2 targeted and KO alleles are crossed into the C57BL/6 inbred strain. For determination of the growth curve groups, we analysed BICD2 mice (both male and female mice) of different genotypes every 2 days from birth to 21 days of age at fixed time points during the day. In addition to the homemade BICD2-deficient mice, we used in this study transgenic mice expressing Nestin-Cre [14] (Jackson Laboratory), EMX1-Cre [16] (Jackson Laboratory), Math1-CreERT2 (ref. 23 ) (Jackson Laboratory), GFAP-Cre [15] (Jackson Laboratory) and GFAP-GFP transgenic mice (kindly provided by Frank Kirchhoff). Information about the mouse lines can be found in the Jackson Laboratory mouse database ( http://jaxmice.jax.org ). Generation of BICD2-deficient mice Targeting techniques and the procedures for selection of ES cells and generation of KO mice have been described [53] . We introduced the resistance markers in ES cells by two sequential rounds of homologous recombination (first round, neomycine cassette, 4.2% (9 out of 213) of picked clones targeted; second round, puromycine cassette, 0.3% (1 out 350) of the picked clones targeted). To test if Cre-mediated excision occurs within the BICD2 locus, we electroporated ES cells with a construct containing the Cre recombinase gene, driven by a thymidine kinase promoter, in a vector backbone with a Pgk hygromycin-resistance gene. After selection with hygromycin B, we detected the deletion of the BICD2 region between the outermost loxP sites by PCR analysis using primer a/d. The positive ES cell clone that was able to excise the BICD2 locus and contains a correct karyotype, was injected into blastocysts. The chimeras that gave germline transmission were mated into the C57BL/6 background to generate inbred Bicd2 f (targeted) mice. Heterozygous BICD2 KO ( Bicd2 − ) mice were obtained by crossing F1 heterozygous Bicd2 f mice with CAG-Cre transgenic mice that express Cre recombinase in the germ-cell lineage (kindly provided by Frank Grosveld). We determined the genotypes of the heterozygous and homozygous Bicd2 f and Bicd2 − mice by PCR analysis using the primer sets indicated in Supplementary Fig. 1A . PCR primers used are primer-a (5′-GTGTAGCACTTCAGGAACATCCATGC-3′), primer-b (5′-AATGGAGAAGATCTCATCTTGGCAGG-3′), primer-c (5′-CGGCGGCATCAGAGCAGCCGATTG-3′) and primer-d (5′-TGTCAGCAAACTCCATCTCTAGCCTC-3′). Western blot analysis using homemade anti-rabbit BICD2 antibodies [4] confirmed the lack of BICD2 protein in brain lysates of P20 Bicd2 −/− mice. To obtain nervous-system-specific KO of BICD2, Bicd2 f/f mice were crossed with transgenic mice expressing Cre recombinase under control of the Nestin promotor [14] (Jackson Laboratory). To examine the role of BICD2 in excitatory neurons in the cortex/hippocampus and premigratory granule cells in the cerebellum, Bicd2 f/f mice were crossed with EMX1-Cre [16] (Jackson Laboratory) and Math1-CreERT2 transgenic mice [23] (Jackson Laboratory), respectively. To obtain sustained expression of Cre-recombinase in astrocytes, including Bergmann glia cells, Bicd2 f/f mice were crossed with GFAP-Cre transgenic mice [15] (Jackson Laboratory). Wild-type and Bicd2 KO mice were also crossed with GFAP–GFP transgenic mice, to visualize the morphology of GFP-labelled Bergmann glia cells [54] (kindly provided by Frank Kirchhoff). The primer sets for PCR genotyping of the various transgenice mouse lines used in this study are described in the Jackson Laboratory mouse database ( http://jaxmice.jax.org ). Histological procedures Mice were anesthetized with pentobarbital and perfused transcardially with 4% paraformaldehyde, and brains were either embedded in paraffin and sectioned at 4–6 μm, or incubated with increasing concentrations of sucrose (15% and 30%) and rapidly frozen and sectioned at 40 μm (freezing microtome) and collected in PBS. Sections were stained with haematoxylin/eosin (paraffin sections), thionin (frozen sections), processed for LacZ staining or processed for immunohistology. For LacZ staining sections were washed with PBS and incubated overnight at 37 °C in PBS buffer containing 1 mg ml −1 X-gal, 5 mM K 3 Fe(CN) 6 , 5 mM K 4 Fe(CN) 6 , 2 mM MgCl 2 , 0.01% SDS and 0.02% NP-40, washed, mounted on glass slides, and counter stained with Neutral Red. For double and triple-labelling immunofluorescence, we used a two-step procedure with FITC-, cyanine 3 (Cy3)-, Cy5-, Alexa Fluor488-, Alexa Fluor468- and Alexa Fluor633-conjugated secondary antibodies (Jackson ImmunoResearch, West Grove, PA; Invitrogen) diluted at 1:400 (see also Supplementary Methods ). For immunohistochemistry, we used an avidin-biotin–immunoperoxidase complex method (ABC; Vector Laboratories) with diaminobenzidine (0.05%) as the chromogen, and biotinylated secondary antibodies (Jackson ImmunoResearch, see Supplementary Methods for details). Primary antibodies used in this study are as follows (see also Supplementary Methods for details): rabbit anti-BICD2 (Ab 2293 and 2294) [4] ; mouse anti-calbindin (Sigma, clone CB-955, 1:10,000); rabbit anti-calbindin (Swant, 1:10,000); guinea pig anti-EAAT2 (Millipore, 1:5,000); goat anti-FoxP2 (AbCam, 1:1,000); rabbit anti-α6GABA A receptor (Sigma, 1:1,000); rabbit anti-GFAP (DAKO, 1:5,000); mouse anti-GFAP (Sigma, clone G-A-5, 1:10,000); mouse anti-mGluR2 (AbCam 1:1,000); mouse anti-NeuN (Millipore MAB377, 1:2,000); mouse anti-neurofilament-M (Sigma, 1:10,000); mouse anti-parvalbumin (Sigma, 1:10,000); mouse anti-Rab6 (ref. 7 ), rabbit anti-Tenascin-C (GeneTex, 1:400), guinea pig anti-VGluT1 (Millipore, 1:2,000), guinea pig anti-VGluT2 (Millipore, 1:1,000) and mouse-anti-MAP2 (Sigma, 1:2,000). Sections stained for immunofluorescence were analysed with Zeiss (Oberkochen, Germany) LSM 510 or LSM700 confocal laser scanning microscopes using 40 × /1.3 and 63 × /1.4 oil-immersion objectives. Immunoperoxidase-stained sections were analysed and photographed using a Leica DM-RB microscope and a Leica DC300 digital camera. Electroporation-mediated transfection of egl cells Rat pups were decapitated at P10, the brain was isolated and placed in ice-cold Leibovitz 15 (L15; Invitrogen) medium. The cerebellum was dissected and meninges removed. The most superficial layer (EGL) of the cerebellum was injected at multiple locations to infuse the cerebellar surface with DNA solution (PBS with 0.02% Fast Green, 400 ng μl −1 pSuper vector, 200 ng μl −1 eGFP vector). The cerebellum was placed between Genepaddles (5 × 7 mm) of a BTX ECM 830 Electroporator and 5 pulses of 87 V for 50 ms with 1.0 s intervals were applied. After electroporation, sagittal slices of 350 μm were cut using a Tissue Chopper (McIlwain). Slices were cultured on inserts (Millipore, 0.4 mm) incubated in culture medium (50% Earls Basal Medium, 25% HBSS, 25% Normal Horse Serum, 5 mM L -glutamine and Penicillin/Streptomycin) for 4 days at 35 °C with 5% CO 2 . Slices were fixed at DIV4 in 4% paraformaldehyde in PBS overnight at 4 °C. Then slices were blocked for 6 h in blocking buffer (5% Normal Goat Serum, 1% BSA, 1% glycine and 0.4% Triton-X100 in PBS) and incubated with primary rabbit anti-GFP antibody (Abcam; 1:2,000) in blocking buffer overnight at 4 °C. Following three washes in PBS, slices were incubated in secondary goat anti-rabbit antibody (Invitrogen; Alexa 488, 1:750) in blocking buffer overnight at 4 °C. To visualize tissue structure, nuclei were stained with 4′,6-diamidino-2-phenylindole. GFP-positive cells were imaged using an Olympus Fluoview FV1000MPE confocal microscope (20 × objective). The number of GFP-positive granule cells in each cerebellar layer was quantified with ImageJ (EGL, molecular/migratory layer and IGL). The fraction of GFP-positive granule cells was calculated for each layer per picture. Three separate experiments were performed (total number of pictures analysed for shScrambled=40, shBicd2=33). Preparation of tissue extracts and mass spectrometry analysis For tissue western blots, total brain, cortex, cerebellum, kidney, lung, spleen, liver and heart were dissected from P20 wild-type, Bicd2 +/− and Bicd2 −/− mice and placed in ice-cold PBS, pH7.4. For developmental western blots, wild-type E10.5 (whole embryo), E13.5, E16, E18, P1, P5 (head only), P10, P15 and adult (cortex and cerebellum) mice were placed in ice-cold PBS, pH 7.4. Samples were homogenized in homogenization buffer (150 mM NaCl, 50 mM Tris, 0.1% v/v SDS, 0.5% v/v NP-40, pH8, 1 × complete protease inhibitors; Roche), briefly sonicated, 10 min centrifuged at 900 rcf, resuspended in SDS sample buffer and boiled for 5 min. Protein concentrations were measured using a BCA protein assay kit (Pierce) and 20 μg of protein was loaded in each lane for a subsequent western blot analysis using standard protocols. For mass spectrometry analysis, the cerebellum was dissected from P15 wild-type and homozygote Bicd2 −/− mice, homogenized, centrifuged and proteins were separated on a 4–12% NuPAGE Bis-Tris gel and stained with the Colloidal Blue staining kit (Invitrogen). Gel lanes were cut into 2-mm slices using an automatic gel slicer and subjected to in-gel reduction with dithiothreitol, alkylation with iodoacetamide and digestion with trypsin as described previously [8] . The Mascot score cutoff value for a positive protein hit was set to 100. Individual peptide tandem mass spectrometry spectra with Mascot scores below 100 were checked manually and either interpreted as valid identifications or discarded. Proteins present in the negative controls (pull-down assays with bio-GFP alone) were regarded as background. For the proteome analysis of the wild-type and homozygote Bicd2 −/− , we focussed on proteins that were previously found to influence neuronal migration, including signalling factors, extracellular matrix and adhesion molecules [24] , [25] , [26] . We searched four mass spectrometry data sets (two from wild-type and two from Bicd2 −/− animals) for the corresponding Mascot score to determine probability of a positive hit and calculated the ratio of wild-type versus KO ( Supplementary Data 1 ). How to cite this article: Jaarsma, D. et al. A role for Bicaudal-D2 in radial cerebellar granule cell migration. Nat. Commun. 5:3411 doi: 10.1038/ncomms4411 (2014).